Chemical sensing with switchable transport channels in graphene grain boundaries Grain boundaries can markedly affect the electronic, thermal, mechanical and optical properties of a polycrystalline graphene. While in many applications the presence of grain boundaries in graphene is undesired, here we show that they have an ideal structure for the detection of chemical analytes. We observe that an isolated graphene grain boundary has ~300 times higher sensitivity to the adsorbed gas molecules than a single-crystalline graphene grain. Our electronic structure and transport modelling reveal that the ultra-sensitivity in grain boundaries is caused by a synergetic combination of gas molecules accumulation at the grain boundary, together with the existence of a sharp onset energy in the transmission spectrum of its conduction channels. The discovered sensing platform opens up new pathways for the design of nanometre-scale highly sensitive chemical detectors. Topological defects improve the sensitivity of carbon-based chemical sensors towards gas molecules due to an efficient physisorption and enhanced charge transfer process [1] , [2] , [3] , [4] , [5] , [6] , [7] . Since such defects are formed within a single-crystalline graphene lattice, they have a modest effect on the electronic properties of the device. Grain boundaries (GBs) in graphene are different as they are formed between misoriented crystalline grains, which can potentially give rise to electronic transport gaps [8] . The emergence of transmission gaps in graphene GBs can be employed to acquire an on/off-like behaviour for the passage of charge carriers upon exposure to gas molecules. In this work, we have isolated an individual GB to study the role of this transport gap on the chemical response of GBs, and observed an ultra-high sensitivity towards adsorbed molecules. We also extended our studies to polycrystalline graphene sensors, and demonstrated the inherent limitation of these sensors compared with individual GBs. Characterization of individual graphene GBs The graphene and GBs used in this study are synthesized using the atmospheric pressure chemical vapour deposition (CVD) technique with precise control over the growth time and environmental conditions [9] , [10] . In this approach, single-crystalline hexagonal graphene grains grow discretely and subsequently coalesce together forming an individual GB ( Fig. 1a ; Supplementary Fig. 1 ). 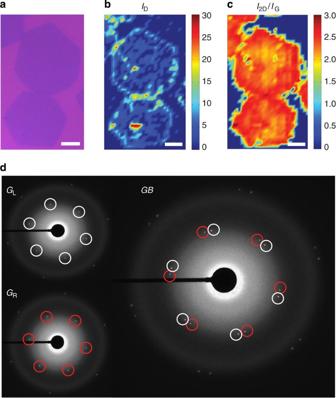Figure 1: Characterization of an individual graphene grain boundary (GB). (a) Optical image of two merged hexagonal graphene grains forming an individual GB (scale bar, 5 μm). (b) D-band Raman mapping of the same graphene grains as shown inFig. 1a. Higher intensity in the merging region of the grains demonstrates the defective nature of the GB. (c) 2D/G ratio mapping of the same region as shown inFig. 1a(Scale bar, 5 μm). The ratio in the range of 2.5 is associated with monolayer graphene. (d) Selected area electron diffraction (SAED) patterns obtained from left (GL), right (GR) grains and the GB region. Sharp and single hexagonal shape evidences the single-crystalline structure of grains. A pattern with two discrete sets of rotated spots appears in the merging region indicating the imperfect stitching of the two graphene grains, which is caused by the crystallographic misorientation across the GB. Figure 1b shows the spatially resolved Raman spectroscopy map obtained for the disorder-induced D band (wavenumber ~1,350 cm −1 ). An intense I D signal obtained in the merging region of the grains provides a strong evidence for the defective nature of the GB region. The occasional I D signals at grains show some structural defects within the perfect lattice, which can be attributed to the nucleation points [10] , [11] . We also mapped the ratio of 2D- to G-band intensity ( I 2D / I G ) where the high intensity ratio (>2.5) all over the scanned area confirms the uniform existence of monolayer graphene ( Supplementary Fig. 2 ). Figure 1d shows selected area electron diffraction patterns obtained from transmission electron microscopy (TEM) for both grains and GB regions. Identical and sharp hexagonal diffraction patterns recorded for the grains in different regions confirm their single-crystalline nature [12] . However, a twofold diffraction pattern was observed when the aperture was located exactly at the merging region disclosing a crystallographic mismatch between the grains, another evidence for the existence of a GB. In addition, high intensity ratio of the {1100} to the {2110} diffraction peaks ( I {1100} / I {2110} ≈1.4) further verifies the existence of monolayer graphene ( Supplementary Fig. 3 ). Figure 1: Characterization of an individual graphene grain boundary (GB). ( a ) Optical image of two merged hexagonal graphene grains forming an individual GB (scale bar, 5 μm). ( b ) D-band Raman mapping of the same graphene grains as shown in Fig. 1a . Higher intensity in the merging region of the grains demonstrates the defective nature of the GB. ( c ) 2D/G ratio mapping of the same region as shown in Fig. 1a (Scale bar, 5 μm). The ratio in the range of 2.5 is associated with monolayer graphene. ( d ) Selected area electron diffraction (SAED) patterns obtained from left (G L ), right (G R ) grains and the GB region. Sharp and single hexagonal shape evidences the single-crystalline structure of grains. A pattern with two discrete sets of rotated spots appears in the merging region indicating the imperfect stitching of the two graphene grains, which is caused by the crystallographic misorientation across the GB. Full size image Chemical-sensing performance of individual GBs We study the chemical-sensing characteristics of individual GBs by monitoring the resistance change of a GB region during the exposure to gas molecules and comparing it with that observed in the gas-exposed grains. All the sensing experiments were performed in ambient conditions using the pulse injection method. 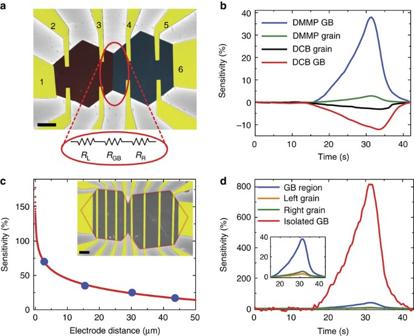Figure 2: Sensing properties of an individual graphene grain boundary (GB). (a) False-colour SEM image of a typical fabricated GB-sensing platform (scale bar, 5 μm). A corresponding electrical circuit is also shown. (b) Sensing signal for the dimethyl methylphosphonate (DMMP) and 1,2-dichlorobenzene (DCB) gas molecules. (c) Fabricated multi-electrodes single-GB-sensing platform (scale bar, 5 μm) and the sensitivity of the GB devices with respect to the distance from the electrodes. (d) Sensitivity of the isolated GB against DMMP molecules extracted from the real-time sensing measurements. The inset magnifies the same curves. Figure 2a shows the false-colour scanning electron microscopy (SEM) image of a typical individual GB-sensing platform. The fabricated structure can be classified in two different regions: single-crystalline grains (further noted as grain) and the GB region (area between electrodes 3 and 4 in Fig. 2a ). The GB region of the device comprises an isolated GB and two trapezoid-shaped grains on the sides. Our sensing platform enabled us to record the simultaneous sensing responses for the left grain, right grain and GB region. A known concentration (50 p.p.b.) of gas molecules (dimethyl methylphosphonate (DMMP) and 1,2-dichlorobenzene (DCB)) were injected over the sensing devices ( Supplementary Fig. 4 ). DMMP and DCB analytes are purposefully selected owing to their electron-donating and -accepting features, respectively. Figure 2b shows the typical sensing response towards DMMP and DCB molecules for grains and the GB region. Here, sensitivity ( S ) is defined as S =( R − R 0 )/ R 0 , where R 0 and R are the initial and final resistance (after gas exposure), respectively. Positive and negative signals upon injection of gas molecules were gained from all the 15 devices tested against DMMP and DCB molecules, in agreement with their electron-donating or -accepting nature [13] . The sensitivity in the GB region (between electrodes 3 and 4) of all the devices is significantly higher compared with the grains’ sensitivity, regardless of the type of gas molecules. For DMMP, the sensitivity of the GB sensors (39.5%) is >1 order of magnitude (14 times) higher than that of grain sensors (2.8%). Similar trend has also been observed for DCB molecules, where the sensitivity of GB sensors (11%) is almost five times higher than in the grain sensors (2.3%). Clearly, the individual GB is responsible for the enhanced sensitivity in the GB region ( Supplementary Note 1 ). Figure 2: Sensing properties of an individual graphene grain boundary (GB). ( a ) False-colour SEM image of a typical fabricated GB-sensing platform (scale bar, 5 μm). A corresponding electrical circuit is also shown. ( b ) Sensing signal for the dimethyl methylphosphonate (DMMP) and 1,2-dichlorobenzene (DCB) gas molecules. ( c ) Fabricated multi-electrodes single-GB-sensing platform (scale bar, 5 μm) and the sensitivity of the GB devices with respect to the distance from the electrodes. ( d ) Sensitivity of the isolated GB against DMMP molecules extracted from the real-time sensing measurements. The inset magnifies the same curves. Full size image We uncovered that the sensing response of an individual GB is significantly improved as the GB is more isolated from its adjacent grains (that is, the electrodes are patterned closer to the GB). In more detail, we fabricated a sensing platform having several electrodes located at different distances from the GB (inset of Fig. 2c ). As shown in Fig. 2c , the GB region sensitivity increases from 17 to 70% (with 50 p.p.b. of DMMP) as the distance between the active electrodes reduces from 43.6 to 2.8 μm. The extension of a fitted exponential curve reveals that a much higher sensitivity may be observed by minimizing the distance between the patterned electrodes. However, single-crystalline graphene grain-based sensors do not show any noticeable length dependency ( Supplementary Fig. 5 ). Note that the device-level sensitivity of the GB-based sensor represents in fact the variation in the overall resistance of GB and the surrounding grain regions (two trapezoid-shaped grains). To exclude the contribution of adjacent graphene regions, a simultaneous sensing experiment was carried out on the left and right grains and GB regions ( Supplementary Fig. 6 ). We measured sheet resistances of the left and right grains ( R □2-3 and R □4-5 ) to calculate the resistance of the adjacent trapezoid-shaped grains ( R TL and R TR in Fig. 2a ). Then, we solved for the additional resistance in the GB region using an equivalent resistance model ( R GB =R 3-4 −(R TL +R TR )) [14] . In absence of any gas molecules, the sheet resistance of ~740Ω/□ was observed for the GB region of the device shown in Fig. 2a (between electrodes 3 and 4) while slightly lower values of 680 Ω/□ and 695 Ω/□ were recorded for the left and right grains, respectively ( Supplementary Fig. 7 ). The higher sheet resistance in the GB region is due to enhanced scattering at GB defect sites [15] . In our devices, the calculated R GB before exposure to gas molecules are found in the range of 5–35 Ω. For the device shown in Fig. 1a , we observed that R GB changed from 15.3 to 142 Ω upon exposure to 50 p.p.b. of DMMP gas molecules. Figure 2d shows the time-dependent sensitivity of the isolated GB, demonstrating a maximum of 828%, which is ~300 times higher compared with the adjacent single-crystalline grains under identical experimental conditions. Such high sensitivity is not observed if the GB is mounted parallel to the direction of charge carrier flow, since lower-resistance pathways around the GB can effectively short-circuit the GB ( Supplementary Fig. 8 ). Comparison with polycrystalline graphene film To investigate the role of GBs in large-area polycrystalline graphene sensors, it is essential to understand the performance of GB sensors as the number of GBs increases. In this regard, we investigated the sensing response of a sequence of multiple GBs, naturally formed by the merging of the grains in the CVD growth. 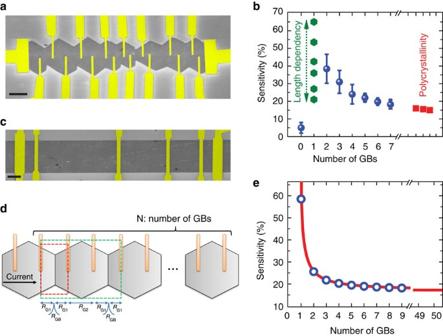Figure 3: Sensitivity versus number of GBs. (a) A typical fabricated multiple GB (7 GBs)-sensing platform (Scale bar, 10 μm). (b) A large-area polycrystalline graphene sensing device (Scale bar, 20 μm). (c) Variation in the sensitivity with respect to the number of GBs, zero represents a single-crystalline flake. The average sensitivity with respect to the number of GBs tends towards the data obtained from large-area polycrystalline sensor. (d) Schematic of the device with multiple GBs used to model the sensitivity cross-over. Equivalent electrical resistance model for multiple graphene GB sensors is also shown. The unit cell is similar to the device shown inFig. 2a. (e) Calculated sensitivity of a multiple GB device as a function of number of GBs. The typical experimental values are plugged into the mathematical model to obtain quantitative results. Figure 3a shows the false-colour SEM image of a typical device with seven GBs. By performing extensive sensing experiments on several devices, we found that the sensitivity drops from 38.9 to 19.8% as the number of GBs increase from 2 to 7. For the case of one GB, a strong length dependency was observed as discussed earlier ( Fig. 2c ), while this dependency becomes less significant in multiple GB devices. We have also fabricated a large-area polycrystalline graphene GB-sensing device containing many GBs ( Fig. 3b ) and performed sensing experiments in similar conditions. We observed a clear sensitivity cross-over from a single GB towards a polycrystalline sensor, as the number of GBs are increased from one to more than five. The results (in Fig. 3c ) show that the sensitivity of multiple GBs sensors approaches the polycrystalline graphene sensitivity (~15%). This behaviour is explained using an equivalent resistance model with a repeating unit cell having similar configuration to the fabricated single-GB device ( Fig. 2a ). In this model, the sensitivity can be represented as: Figure 3: Sensitivity versus number of GBs. ( a ) A typical fabricated multiple GB (7 GBs)-sensing platform (Scale bar, 10 μm). ( b ) A large-area polycrystalline graphene sensing device (Scale bar, 20 μm). ( c ) Variation in the sensitivity with respect to the number of GBs, zero represents a single-crystalline flake. The average sensitivity with respect to the number of GBs tends towards the data obtained from large-area polycrystalline sensor. ( d ) Schematic of the device with multiple GBs used to model the sensitivity cross-over. Equivalent electrical resistance model for multiple graphene GB sensors is also shown. The unit cell is similar to the device shown in Fig. 2a . ( e ) Calculated sensitivity of a multiple GB device as a function of number of GBs. The typical experimental values are plugged into the mathematical model to obtain quantitative results. Full size image where N is the number of GBs, R GB is the resistance of the isolated GB, R G1 is the resistance of the trapezoid-shaped grain region and R G2 is the resistance of the single-crystalline region (shown in Fig. 3d ). The sensitivity of the model as a function of N is calculated using the typical experimental values of the single-GB device, where the sensitivity of the polycrystalline sensor is anticipated to be around 17%, fairly close to the experimental result (15%). For the case of one GB, R G2 is eliminated, thus the sensitivity is greatly increased. The slight difference between the experimental data ( Fig. 3c ) and the calculations ( Fig. 3e ) is due to the asymmetric nature of the fabricated devices ( Fig. 3a ) in terms of variation in the position of the electrodes with respect to GBs, and non-equal resistances of the GBs and the grain regions. However, both results are consistently suggesting that the sensitivity is greatly suppressed as one moves towards polycrystallinity. Notice that in the case of an individual GB, the sensing response can be amplified as the GB becomes more isolated, approaching the very large sensitivity shown in Fig. 2c (828%). However, this is not the case in devices having >1 GB, since the resistance of the grain regions ( R G2 ) between two GBs cannot be avoided. This demonstrates the inherent limitation of the polycrystalline graphene sensors compared with an individual GB sensor with a high degree of isolation. To reveal the microscopic nature of the observed ultra-high sensitivity, we model the electronic structure and transport in a typical GB with an 18° mismatch angle ( Fig. 4a,b ). The GB model consists of a quasi-periodic meandered line of defects formed between two graphene grains (consistent with previous TEM studies [16] ), which are deposited on an amorphous SiO 2 substrate to obtain their realistic doping ( Supplementary Fig. 9 ; Supplementary Note 2 ). We found that the stress-relaxed structure forms a corrugation along the GB with different equilibrium heights from the substrate, giving rise to an effective p – p′–p doping distribution ( Fig. 4c ). The presence of local doping has been demonstrated by calculating a two-dimensional (2D) electrostatic potential profile ( Fig. 4c ) in the GB region, revealing a potential well with large electric field gradients on its sides. Our simulations show that DMMP molecules with a permanent dipole are attracted to the regions of high electric field gradient present at the p – p′–p interface. The accumulation of DMMP molecules at GB results in a local charge donation and modification of the doping distribution ( p — p′′–p ). These results are illustrated in Fig. 4d presenting a one-dimensional potential obtained by averaging of the 2D potential along the direction normal to the GB (with and without DMMP molecules). 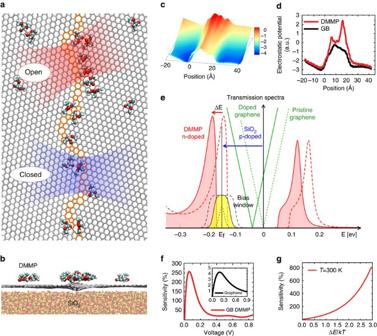Figure 4: Classical and quantum simulation studies. (a) The top and (b) side views of the modelled graphene grain boundary structure deposited on the defective amorphous SiO2substrate with physisorbed DMMP molecules. Two transmission regions with different translational vectors are highlighted in red (small gap) and blue (large gap) colours. (c) Two-dimensional electrostatic potential energy profile across the GB. (d) One-dimensional potential profiles (with and without DMMP molecules) obtained by averaging of the 2D potential along the direction normal to the GB. (e) Calculated transmission spectra (red curves) for the open GB region (highlighted in red inFig. 3a) and the grain region (green dashed line), shown both without and with homogeneous n-doping (green solid line) by DMMP molecules (same adsorbents surface density). The Fermi level,Ef, is shifted down (Dirac point of the grains) due to the p-doping by SiO2. Bias window intersects spectra of certain transmission regions and opens the passage of electrons through them, while adsorbed DMMP molecules tend to close these passage regions. (f) Calculated sensitivity for the GB and graphene grain (inset) with respect to the applied voltage for DMMP molecules. (g) Maximum sensitivity calculated as a function of a DMMP-induced spectral shift over a thermal energy, ΔE/kT. Figure 4: Classical and quantum simulation studies. ( a ) The top and ( b ) side views of the modelled graphene grain boundary structure deposited on the defective amorphous SiO 2 substrate with physisorbed DMMP molecules. Two transmission regions with different translational vectors are highlighted in red (small gap) and blue (large gap) colours. ( c ) Two-dimensional electrostatic potential energy profile across the GB. ( d ) One-dimensional potential profiles (with and without DMMP molecules) obtained by averaging of the 2D potential along the direction normal to the GB. ( e ) Calculated transmission spectra (red curves) for the open GB region (highlighted in red in Fig. 3a ) and the grain region (green dashed line), shown both without and with homogeneous n-doping (green solid line) by DMMP molecules (same adsorbents surface density). The Fermi level, E f , is shifted down (Dirac point of the grains) due to the p-doping by SiO 2 . Bias window intersects spectra of certain transmission regions and opens the passage of electrons through them, while adsorbed DMMP molecules tend to close these passage regions. ( f ) Calculated sensitivity for the GB and graphene grain (inset) with respect to the applied voltage for DMMP molecules. ( g ) Maximum sensitivity calculated as a function of a DMMP-induced spectral shift over a thermal energy, Δ E / kT . Full size image We can split the GB, known to be meandered and otherwise imperfect, into local regions with different transport properties, determined by the crystallographic orientation of the graphene grains, the local angle of GB with respect to the grains and the local topologies of GB defects [8] , [17] . Such regions can form individual electron transport channels with local transmission spectra (gaps) ( Fig. 4a ). Depending on the local doping from the substrate (shift of transmission spectra), these transport channels can be initially either opened or closed. Upon adsorption of electron-donating or -accepting analytes at the GB, the transmission spectra of the channels can be shifted with respect to the Fermi level ( p – p′′–p ). This can open or close some of the electron transport channels, with a potentially large effect on the GB resistance. To illustrate these phenomena, we have calculated the local electron transmission through two selected regions of the GB (shown in Fig. 4a ), with different local angles and defect topologies ( Supplementary Figs 9 and 10 ). We found that the transport of electrons with energies close to E f is strongly suppressed resulting in transport gaps ( Supplementary Fig. 11 ). The transmittance reveals very different transport gaps (~0.2 eV, ~1 eV) for the two GB regions ( Supplementary Notes 2 and 3 ). We assume that only regions with the smallest energy gaps and energy onsets can significantly contribute to the molecular sensing. Note that graphene GBs feature isolated states near E f [8] , [15] , [17] , [18] , [19] , [20] , [21] , [22] . However, these spatially localized states are not visible in the GB transmissivity, since they do not overlap with the electrode states. Figure 4e shows the equilibrium transmission spectrum through the low-gap (0.2 eV) region before (red-dashed curve) and after (red-shadowed curve) adsorption of DMMP molecules. Since the graphene subsystem is p-doped by SiO 2 ( Supplementary Fig. 12 ), E f (thin black line) in Fig. 4e is shifted downwards (by ~0.15 eV, Supplementary Notes 3 and 4 ) from the zero-level energy (non-doped case). In the presence of DMMP, GB is additionally n-doped, as shown by a shifted transmission spectrum down (by ~0.05 eV) with respect to E f , assuming that E f stays fixed with respect to the rest of the system (grains transmission spectra shown by green dashed lines). The 0.05 eV shift corresponds to an electron density concentration of ~2.5 × 10 11 cm −2 , which is compatible with DMMP/graphene experimental values [23] . We used these two spectra to calculate an electron current passing through the GB region under bias (yellow area in Fig. 4e ) in the presence and absence of homogenously distributed DMMP molecules (Supplementary Note 3). We schematically show the bias window (yellow area in Fig. 4e ) positioned around E f . One can see that for the p-doped system the current flow passes (windows overlap with GB spectrum), while when DMMP n-dopes GB, the current does not flow (no overlap) unless bias is increased enough ( Supplementary Fig. 13 ). Figure 4f presents the obtained bias-dependent sensitivities ( Supplementary Equations 1 and 2 ) for DMMP analytes for both GB (channel region) and pristine graphene (inset figure) under the same doping conditions (substrate and density of DMMP), showing a prominent sensitivity peak, in agreement with our experiments ( Supplementary Fig. 14 ). The used transmission spectra are shown by red and green lines in Fig. 4e (pristine graphene needs more exposure to the adsorbants for the same DMMP surface density). Because of the sharp transmission onset of the GB transport channel ( Fig. 4e ), the calculated maximum sensitivity (250%) is 60 times larger than that of graphene (4%). Using a simplified analytical model ( Supplementary Equation 3 ), we have performed additional calculations to find how the maximum sensitivity of the GB device depends on the transmission spectra shift, Δ E , caused by the local adsorption of analytes ( Fig. 4g ). We found that an n-doping shift of 0.08 eV≈3 k B T is required to achieve the ~800% experimentally observed sensitivity. This shift of the GB spectrum seems to be realistic due to the additional accumulation of the DMMP molecules adsorbed around the GB ( Fig. 4d ). The presented sensing mechanism has an inherent symmetry for electron-donating and -accepting analytes. To obtain maximum sensitivity for each case, the Fermi level should be tuned by gate doping closely below (above) the energy onset for the electron donors (acceptors), hence they can close (open) the electron transport channels. In summary, we have investigated the gas-sensing behaviour of GBs present in graphene. It was shown that the sensitivity of an isolated GB is ~300 times higher than that of a single graphene grain and much larger than that of polycrystalline graphene sensors. We have verified that the presence of local transport gaps in GBs together with the local accumulation of gas molecules plays a crucial role in the observed large chemical sensitivity of GBs, so the mechanism differs from the previously reported carrier density modulation in carbon-based sensors [6] , [7] , [23] , [24] , [25] , [26] , [27] , [28] . The sensing mechanism is based on a marked closing or opening of local conduction channels through the GB by the adsorbed analytes. This new sensing modality can be used to develop real nanometre-scale sensors with numerous potential applications. Graphene growth Graphene GBs were synthesized on copper foils (from Alfa Aesar, product no. 46365) by the CVD process at ambient pressure [9] , [10] . At first, copper foils were treated for 10–20 min in hydrochloric acid (10% diluted in deionized water) and rinsed properly in acetone and isopropanol followed by drying in argon (Ar) gas flow to clean the surface. The cleaned samples were immediately loaded into the CVD chamber. After loading the samples, first, the CVD chamber was evacuated (down to 1 mtorr) and then purged with forming gas (5% hydrogen diluted in Ar) up to the atmospheric pressure. The samples were heated up to 1,050 °C in protection of forming gas and annealed for 60 min. Annealing in H 2 helps in improving the Cu surface quality by reducing the concentration of nucleation points. Finally, the graphene growth was carried out by introducing 20 p.p.m. of methane (CH 4 ) for a precisely controlled time (for example, 50 min) to obtain the desired grain size and surface coverage. The samples were then rapidly cooled down to room temperature in protection of forming gas and carefully taken out for further procedure. Raman spectroscopy The Raman spatially resolved maps were obtained using a Horiba JobinYvonXplora confocal Raman microscope equipped with a motorized sample stage from Marzhauser Wetzlar. The laser excitation wavelength was 532 nm and the maps were obtained for graphene GB samples transferred on SiO 2 substrate. The spectral resolution of the laser was 2.5 cm −1 , and pixel size of the map was 500 nm. D (~1,350 cm −1 ), G (~1,580 cm −1 ) and 2D-band (~2,690 cm −1 ) spatial maps were extracted. TEM TEM images and diffraction patterns were acquired on an aberration-corrected JEOL JEM-ARM200CF, operated at 80 kV to avoid the beam damage effects. At first, graphene samples were transferred to a 30-nm-thick Silicon Nitride membrane using a polymer-assisted transfer technique. Further, samples were annealed at 350 °C for 3–4 h in the presence of forming gas (5% H 2 in Argon) to clean the residual contamination and then the sample grid was loaded into the microscope for characterization. SEM SEM was performed to visualize the morphology of the GB-sensing devices. The instrument used for characterization is integrated in a Raith e-LiNE plus ultra-high-resolution electron beam lithography system. We used the acceleration voltage of 4 and 10 kV for imaging before device fabrication and after sensing experiments, respectively. The current was also minimized by reducing the aperture size to decrease the electron beam-induced defects. No particular types of preparation were implemented before imaging the GB devices. Device fabrication The grown graphene films (on Cu) with distinguishable GBs were transferred to a highly doped Si/SiO 2 wafer, using the poly(methyl methacrylate) (PMMA)-assisted technique. The transferred GB samples were then annealed in a furnace at 350 °C for 90 min in presence (flow rate −70 s.c.c.m.) of the forming gas (5% H 2 in Ar) to remove the polymer residues. Using the geometrical shape of the flakes in the partially covered graphene film, we were able to detect the GBs and locate them relative to the predefined alignment marks on the substrate. The images obtained from bright-field optical microscopy (or SEM at low acceleration voltage) were used to design the electron beam lithography patterns. In one lithography step, followed by O 2 plasma cleaning, excess of graphene flakes were etched away to remove the electrical pathways between electrodes through undesired graphene flakes. In another step, electrode patterns were transferred onto the sample and chromium/gold (7/50 nm) electrodes were deposited using electron beam evaporation system. We tried to avoid defining the geometry of the sensors to reduce the edge defects and eliminate their corresponding gas-sensing response. We used a bilayer PMMA coating for both of the lithography steps to facilitate the metal lift-off process and obtain higher etch resistance. Before the sensing experiments, the samples were again annealed at 400 °C for 2 h to remove the residues from the fabrication process. Sensing experiments The sensing experiments were performed using a customized sensing platform ( Supplementary Fig. 4 ). In brief, the HP 6890 gas chromatography system was used to inject a known volume (0.2 μl) of DMMP or DCB with 1/5,000 split ratio. DMMP and DCB were purchased from the Sigma-Aldrich and used without any process. Electrical resistances of the devices were monitored using Keithley 2612A source-meter. A constant current (50 μA) was applied across the electrodes during the sensing experiments. Computational details We combine classical and quantum molecular dynamics (MD) simulations to model the graphene GBs deposited on a defective amorphous SiO 2 . The classical MD simulations are performed with NAMD [29] , [30] and the CHARMM32 force field [31] . During our simulations, we keep the temperature fixed at T =300 K by the Langevin dynamics with a damping constant of γ Lang =1 ps −1 . The switching distance for non-bonded interactions is set to 8 Å, and the cutoff is set to 10 Å. The systems are simulated in an NVT ensemble (the ensemble with constant number of particles, constant volume and constant temperature), where the particle mesh Ewald summation [32] is used to describe a long-range Coulombic coupling. In each classical simulation, we first minimize the system energy and then equilibrate the system for ~10 ns at T =300 K. In the quantum MD simulations, we use TeraChem [33] , [34] , [35] with energies and forces evaluated using the Becke, Lee, Yang and Parr exchange-correlation functional with a 3–21-g basis set and charges calculated within the Mulliken scheme ( Supplementary Fig. 9 ). How to cite this article: Yasaei, P. et al. Chemical sensing with switchable transport channels in graphene grain boundaries. Nat. Commun. 5:4911 doi: 10.1038/ncomms5911 (2014).